Hall effect of triplons in a dimerized quantum magnet SrCu 2 (BO 3 ) 2 is the archetypal quantum magnet with a gapped dimer-singlet ground state and triplon excitations. It serves as an excellent realization of the Shastry–Sutherland model, up to small anisotropies arising from Dzyaloshinskii–Moriya interactions. Here we demonstrate that these anisotropies, in fact, give rise to topological character in the triplon band structure. The triplons form a new kind of Dirac cone with three bands touching at a single point, a spin-1 generalization of graphene. An applied magnetic field opens band gaps resulting in topological bands with Chern numbers ±2. SrCu 2 (BO 3 ) 2 thus provides a magnetic analogue of the integer quantum Hall effect and supports topologically protected edge modes. At a threshold value of the magnetic field set by the Dzyaloshinskii–Moriya interactions, the three triplon bands touch once again in a spin-1 Dirac cone, and lose their topological character. We predict a strong thermal Hall signature in the topological regime. Topological phases of bosons have steadily gained interest, driven by the goal of realizing protected edge states that do not suffer from dissipation. As bosonic carriers (phonons, magnons and so on) are electrically neutral, they are weakly interacting and show good coherent transport. As a first step in this direction, analogues of the integer quantum Hall effect have been proposed using photons [1] , [2] , [3] , [4] , magnons [5] , [6] , [7] , [8] , [9] , phonons [10] , [11] , [12] and skyrmionic textures [13] , with the thermal Hall effect [14] as the experimental probe of choice. It would be very interesting to observe this phenomenon in quantum magnets, where the quantization of spin produces a new class of bosonic excitations called triplons. The archetypal quantum magnet is SrCu 2 (BO 3 ) 2 , a layered material consisting of Cu S =1/2 moments arranged in orthogonal dimers [15] , [16] . To a very good approximation, this arrangement conforms to the Shastry–Sutherland model [17] , [18] . Low-energy excitations correspond to breaking a singlet to form a triplet. Such excitations are called triplons and can be thought of as spin-1 bosonic particles [19] . Indeed, triplons undergo Bose condensation in many systems [20] , [21] , [22] . If SrCu 2 (BO 3 ) 2 were an exact realization of the Shastry–Sutherland model, the triplons would be local excitations forming a threefold-degenerate flat band [23] . However, electron spin resonance (ESR) [24] , infrared absorption [25] , neutron scattering [26] and Raman scattering [27] measurements show a weak dispersion that has been attributed to small Dzyaloshinskii–Moriya (DM) anisotropies [28] , [29] , [30] . Nuclear magnetic resonance measurements also support the presence of DM couplings [31] . Here, we show that DM couplings give rise to topological character in the triplon energy spectrum of SrCu 2 (BO 3 ) 2 . A small magnetic field suffices to induce phases with Chern bands and topologically protected edge states. As triplons carry energy but no electrical charge, we predict a thermal Hall effect of triplons. 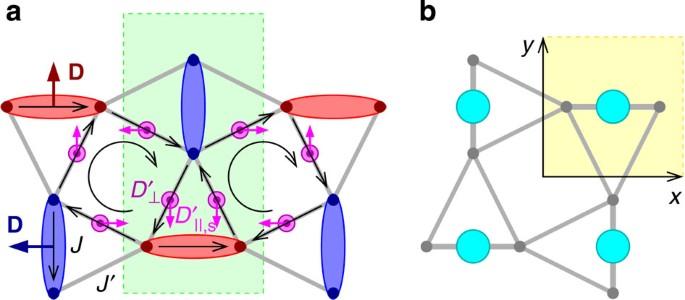Figure 1: The SrCu2(BO3)2lattice. (a) Heisenberg and DM couplings in SrCu2(BO3)2. The red and blue arrows on dimers represent the intra-dimer DM vectorsD(black arrows indicate the order of spins in the DM term). The inter-dimer couplingD′ has in-plane and out-of-plane components. Following the circular arrows as indicated, the out-of-plane DM component points out of the plane (purple circles). The ‘staggered’ in-plane component is shown by magenta arrows. The green rectangle indicates the structural unit cell. (b) The new reduced unit cell upon taking the two dimers to be equivalent is shown in the yellow square. The dimers form a square lattice as shown. Microscopic model Figure 1a illustrates the lattice geometry and the interactions between the spins in SrCu 2 (BO 3 ) 2 . The Hamiltonian is given by Figure 1: The SrCu 2 (BO 3 ) 2 lattice. ( a ) Heisenberg and DM couplings in SrCu 2 (BO 3 ) 2 . The red and blue arrows on dimers represent the intra-dimer DM vectors D (black arrows indicate the order of spins in the DM term). The inter-dimer coupling D ′ has in-plane and out-of-plane components. Following the circular arrows as indicated, the out-of-plane DM component points out of the plane (purple circles). The ‘staggered’ in-plane component is shown by magenta arrows. The green rectangle indicates the structural unit cell. ( b ) The new reduced unit cell upon taking the two dimers to be equivalent is shown in the yellow square. The dimers form a square lattice as shown. Full size image J is the strength of the exchange coupling on intra-dimer bonds. The intra-dimer DM coupling D is allowed by symmetry below a structural phase transition at T ∼ 395 K (refs 32 , 33 ; see Supplementary Figs 1 and 2 , Supplementary Table 1 and Supplementary Note 1 ). We have included a small magnetic field h z perpendicular to the SrCu 2 (BO 3 ) 2 plane, with the g-factor denoted as g z . On the inter-dimer bonds, J ′ and D ′ are the exchange and DM couplings, respectively, with the dominant DM component being out-of-plane. As seen in Fig. 1a , the out-of-plane couplings encode a sense of clockwise rotation; this ultimately drives a Hall effect of triplon excitations as we report below. Triplon description A thorough bond operator treatment of the Hamiltonian in equation 1 has been presented in ref. 30 . We present a simplified treatment suitable for SrCu 2 (BO 3 ) 2 in a weak magnetic field. Previous studies have largely focused on plateau phases at high fields(ref. 34 and references therein). In contrast, we show that the low-field regime has exotic topological properties. In a given dimer, the Hilbert space is spanned by a singlet and three triplets: and . In the pure Shastry–Sutherland model, the ground state is a direct product of singlets | s 〉 over the dimers as long as J ′ ≲ 0.675 J (refs 18 , 35 , 36 ). In SrCu 2 (BO 3 ) 2 , as the DM anisotropies are small compared with J , we assume that the ground state remains a product wavefunction. Minimizing the overall energy, we find that the ground state has the wavefunction and on horizontal and vertical dimers, respectively; the direction of D on each dimer determines whether | t y 〉 or | t x 〉 is admixed. The triplet admixture is proportional to the intra-dimer DM coupling | D | with . Here, as in the rest of this article, we only retain terms up to linear order in D , D ′, and h z , which are small compared with the J ′s. On each dimer, we choose a new Hilbert space by rotating to using on horizontal and vertical dimers, respectively. In the ground state, each dimer is in the state given by the first row in the corresponding W matrix. We have three local excitations given by the mutually orthogonal triplon states , and . At low-magnetic fields, the low-energy excitations are spanned by single-triplon states with their dynamics captured by hopping processes of the form . Introducing a bosonic representation for triplons, we obtain a Hamiltonian with purely hopping-like terms. By defining W v as above with complex entries, the Hamiltonian takes on a convenient form, viz., the two dimers in the unit cell become equivalent (see Supplementary Note 2 for details). We may henceforth drop v / h indices and work with the reduced unit cell in Fig. 1b . In momentum space, the Brillouin zone (BZ) is enlarged as shown in Fig. 2b . 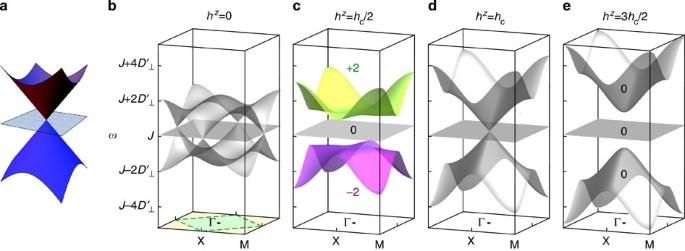Figure 2: Topological transitions in the triplon bands. (a) A spin-1 Dirac cone with three bands touching. (b) Triplon dispersion forhz=0. The basal plane shows the enlarged BZ corresponding to one dimer per unit cell, withk=(π,π) at the M andk=(π,0) and (π,0) at the X points. The smaller structural BZ is shown in green. The band structure hosts spin-1 Dirac cones at the BZ edge centres X. (c–e) Evolution of triplon bands and Chern numbers upon tuning magnetic field. Bands with non-zero Chern number appear for 0<hz<hcand are shown in colour. Athz=hc(d), the bands touch at a spin-1 Dirac cone at Γ. Forhz>hcas ine, the Chern numbers remain zero. Figure 2: Topological transitions in the triplon bands. ( a ) A spin-1 Dirac cone with three bands touching. ( b ) Triplon dispersion for h z =0. The basal plane shows the enlarged BZ corresponding to one dimer per unit cell, with k =( π , π ) at the M and k =( π ,0) and ( π ,0) at the X points. The smaller structural BZ is shown in green. The band structure hosts spin-1 Dirac cones at the BZ edge centres X. ( c – e ) Evolution of triplon bands and Chern numbers upon tuning magnetic field. Bands with non-zero Chern number appear for 0< h z < h c and are shown in colour. At h z = h c ( d ), the bands touch at a spin-1 Dirac cone at Γ. For h z > h c as in e , the Chern numbers remain zero. Full size image For a more complete treatment, we may include pairing-like terms ( ) within a bond operator formalism as in ref. 30 . We ignore such terms as they do not change the triplon energies to linear order in D , D ′ and h z ; we have checked that their inclusion does not alter the results presented here. Spin-1 Dirac cone physics The triplon Hamiltonian in momentum space is given by where the Hamiltonian matrix is given by with γ 1 ( k )=sin k x , γ 2 ( k )=sin k y and (see Supplementary Note 2 for details). Only two components of the inter-dimer DM coupling enter the Hamiltonian, viz., the out-of-plane component and the ‘staggered’ component shown in Fig. 1a . A third non-staggered component is allowed by symmetry, but does not appear at this level (see Supplementary Fig. 2 and Supplementary Note 1 ). Intra-dimer D and in-plane inter-dimer act in consonance so that only the linear combination appears in the Hamiltonian similar to the analysis in ref. 29 . In the following, we use the values J =722 GHz, , and g z =2.28 in the M ( k ) matrix, which reproduce the ESR data in ref. 24 . The parameter J is not the microscopic exchange strength, but rather the measured spin gap, which determines the effective coupling in the presence of quantum fluctuations. The M ( k ) matrix is of the form where 1 is the 3 × 3 identity matrix and is a vector of 3 × 3 matrices satisfying the [ L ξ , L η ]= iɛ ξηζ L ζ SU(2) algebra. Thus, in momentum space, the triplons behave as (pseudo)spin-1 objects coupled to a pseudomagnetic field We now draw an analogy with the usual two-band physics wherein the 2 × 2 Hamiltonian takes the same form as equation (5) but with spin-1/2 Pauli matrices instead of spin-1 L matrices. There, we obtain two bands corresponding to eigenvalues J ± d ( k )/2 (we denote d ( k )=| d ( k )|). If d ( k ) is non-zero throughout the BZ, we obtain two well-separated bands whose Chern numbers are ± N s , where N s is the number of skyrmions in the d ( k ) field over the BZ [37] . The d ( k ) field contains all information about the band structure; its skyrmion count determines the topological character of bands. We emphasize here that topological properties will not change with small corrections to the Hamiltonian such as next-nearest neighbour hopping (see Supplementary Figs 3 and 4 , and Supplementary Note 3 ). Likewise, in our spin-1 realization, we read off the eigenvalues as { J + d ( k ), J , J − d ( k )}. Note that the band in the middle is always flat with energy J , irrespective of the value of d ( k ). If the pseudomagnetic field d ( k ) vanishes at some k , all three bands touch in a ‘spin-1 Dirac cone’, resembling graphene but with an additional flat band passing through the band touching point. If d ( k ) is non-zero throughout the BZ, the spectrum consists of three well-separated triplon bands with well-defined Chern numbers {−2 N s ,0,+2 N s }, where N s is again the skyrmion number. More generally, for the arbitrary spin- S generalization of equation (5), we have (2 S +1) bands with Chern numbers {−2 SN s ,−2( S −1) N s ,…, 2(S−1), 2 SN s } (see Supplementary Table 2 and Supplementary Note 4 ). Magnetic field-tuned topological transitions The magnetic field h z provides a handle to tune topological transitions in SrCu 2 (BO 3 ) 2 , as shown in Fig. 2 . With small magnetic fields, even though the ground state remains a product of dimer singlets, the band structure of excitations shows topological transitions. When h z =0, the three bands touch at the edge centres of the BZ (corresponding to corners in the structural BZ). A small applied field opens a non-trivial band gap, allowing for three well-separated bands with Chern numbers {−2,0,+2} or {+2,0,−2}, depending on the sign of h z . When the field reaches a threshold strength , the three bands touch at the Γ point. Indeed, this band touching has already been seen in ESR [24] and infrared absorption [25] spectra at h z ≈1.4 T; however, its significance as a spin-1 Dirac point was not appreciated. As h z is increased further, a trivial band gap opens with all three Chern numbers being zero. The topology of triplon bands can be understood in terms of the d ( k ) field. To every point in the two-dimensional (2D) BZ (an torus), we assign the 3D vector d ( k ): this gives us a closed 2D surface embedded in three dimensions. If the bands are to remain well-separated, the surface cannot touch the origin, that is, d ( k )≠0 anywhere in the BZ. The origin is thus special and acts as a monopole for Berry phase. The topology of the band structure reduces to whether or not the 2D surface encloses the origin; if it does, how many times does it wrap around the origin? This defines a skyrmion number , that is related to the Chern number. To see the role of h z , we note that it enters solely as an additive contribution in the z-component of d ( k ). As shown in Fig. 3 , the BZ maps to a closed surface of width and height proportional to , which is composed of an upper and a lower chamber. The chambers are disconnected, but touch along line nodes. The surface is orientable: the outer surface of the lower chamber smoothly connects to the inner surface of the upper chamber and vice versa. When | h z |> h c , neither chamber encloses the origin; we have N s =0 with all Chern numbers zero ( Fig. 3a,d ). When − h c < h z <0, the origin lies inside the upper chamber ( Fig. 3b ), the net Berry flux is positive and Chern numbers are {+2,0,−2}. When 0< h z < h c , the origin lies inside the lower chamber ( Fig. 3c ), the Berry flux is negative and Chern numbers are {−2,0,+2}. 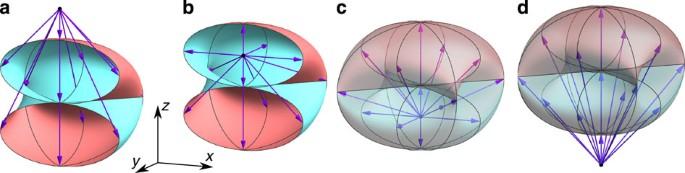Figure 3: Chern numbers from Berry flux. Topological 2D surface obtained from mapping each point in the BZ to a 3Dd(k) vector whenhztakes the values (a) −3hc/2, (b) −hc/2, (c)hc/2 and (d) 3hc/2. The arrows in the figure emanate from the origin, which acts as a monopole of Berry flux. Figure 3: Chern numbers from Berry flux. Topological 2D surface obtained from mapping each point in the BZ to a 3D d ( k ) vector when h z takes the values ( a ) −3 h c /2, ( b ) − h c /2, ( c ) h c /2 and ( d ) 3 h c /2. The arrows in the figure emanate from the origin, which acts as a monopole of Berry flux. Full size image The key ingredient that gives rise to topological properties is the DM interaction that originates from relativistic spin-orbit coupling. The threshold magnetic field h c is proportional to the coupling . The intra-dimer DM coupling D also plays a role: we do not find any Chern bands upon setting D =0, as is appropriate for T >395 K, above a structural transition in SrCu 2 (BO 3 ) 2 . Edge states The topological character of bands is revealed when edges are introduced. For 0< h z < h c (and for − h c < h z <0), edge states connecting the Chern bands appear within the bulk band gap, as shown in Fig. 4a for a strip geometry. Apart from recovering the bulk bands, we clearly see four edge states consistent with bulk boundary correspondence [38] for Chern numbers ±2. The edge states constitute two ‘right-movers’ and two ‘left-movers’ (with group velocity pointing right/left), localized on the opposite edges of the strip. The wave functions of the edge states decay exponentially into the bulk, as shown in Fig. 4b . 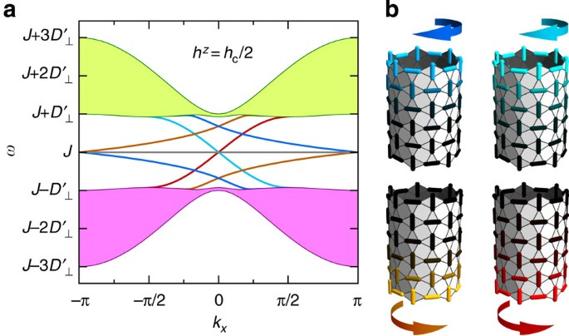Figure 4: Protected edge states. (a) Band structure of SrCu2(BO3)2on a cylindrical strip periodic inx, but with open edges alongy. The width alongyis taken to be very large. We recover the bulk states corresponding to three triplon bands. In addition, four edge states appear, connecting the Chern bands. Edge modes shown in blue and cyan (red and brown) are left-movers (right-movers). (b) Wavefunctions of the four edge states for an arbitrarykxon a strip of widthW=8 dimers. The colour of the dimer bond represents the triplon weight with black corresponding to zero. Right-moving edge states are localized on the bottom edge, whereas left-movers are localized on the top edge. Figure 4: Protected edge states. ( a ) Band structure of SrCu 2 (BO 3 ) 2 on a cylindrical strip periodic in x , but with open edges along y . The width along y is taken to be very large. We recover the bulk states corresponding to three triplon bands. In addition, four edge states appear, connecting the Chern bands. Edge modes shown in blue and cyan (red and brown) are left-movers (right-movers). ( b ) Wavefunctions of the four edge states for an arbitrary k x on a strip of width W =8 dimers. The colour of the dimer bond represents the triplon weight with black corresponding to zero. Right-moving edge states are localized on the bottom edge, whereas left-movers are localized on the top edge. Full size image Thermal Hall effect Chern bands in electronic systems can be easily probed by doping the system so that the Fermi level lies in the band gap. This gives a transverse electrical conductivity quantized to integer values. In bosonic systems where this is not possible, the thermal Hall effect provides an alternative. Semi-classical analysis shows that a wave packet in a Chern band undergoes rotational motion [39] , [40] . To exploit this, a temperature gradient is used to populate the band differently at the system’s edges. The rotational motion of the triplons is then unbalanced, leading to a transverse triplon current. As triplons carry energy, this leads to a measurable transverse thermal current. An expression for thermal Hall conductivity was derived using the Kubo formula in ref. 5 . Subsequently, Matsumoto et al . [7] showed that there is an extra contribution from the orbital motion of excitations. 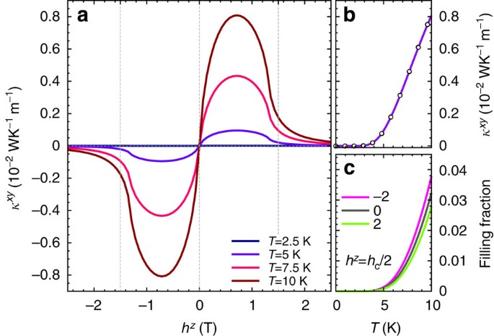Figure 5: Thermal Hall effect. (a) Thermal Hall conductivity versus external magnetic field at different temperatures. The threshold fieldshz=±hcare shown as vertical dashed lines. (b) Thermal Hall signal athz=hc/2 versus temperature. The circles are direct evaluation of the formula, the line is an approximation applicable to SrCu2(BO3)2in the limit where bandwidths are much smaller than the gap. (c) The filling fraction (boson occupation number) for the three bands, indexed by Chern numbers. It grows much slower with temperature thanκxy. Figure 5a shows the thermal Hall conductivity as a function of external magnetic field calculated using the expression in ref. 7 . SrCu 2 (BO 3 ) 2 is quasi-2D and the Hall response in each layer is in the same direction. Therefore, we add the contribution from each layer to get κ xy for a three-dimensional sample ( see Supplementary Note 5 ). As the magnetic field is tuned away from h z =0, a non-zero Hall signal develops with the sign of κ xy depending on the direction of magnetic field. When the threshold magnetic field strength h c is reached, the topological nature of triplon bands is lost and the Hall signal is diminished. Figure 5b shows the peak thermal Hall conductivity increasing monotonically with background temperature. Our calculation assumes that the temperature is low enough that the triplon bands are weakly populated, allowing us to neglect triplon–triplon interactions. We expect this assumption to hold atleast until ∼ 5 K where the filling of bosons is ∼ 0.2%. Neutron scattering data show that the intensity of the single triplet excitations is essentially unchanged up to 5 K showing no damping [26] . Figure 5: Thermal Hall effect. ( a ) Thermal Hall conductivity versus external magnetic field at different temperatures. The threshold fields h z =± h c are shown as vertical dashed lines. ( b ) Thermal Hall signal at h z = h c /2 versus temperature. The circles are direct evaluation of the formula, the line is an approximation applicable to SrCu 2 (BO 3 ) 2 in the limit where bandwidths are much smaller than the gap. ( c ) The filling fraction (boson occupation number) for the three bands, indexed by Chern numbers. It grows much slower with temperature than κ xy . Full size image We have demonstrated that SrCu 2 (BO 3 ) 2 hosts a Hall effect of triplons. A small external magnetic field of the order of a few Tesla suffices to tune topological transitions in the band structure. The triplons form novel spin-1 Dirac cones with threefold band touching. Such a feature has been seen in various contexts [41] , [42] , [43] , [44] , [45] . Our study elucidates its implications for band structure topology; the spin-1 structure naturally gives Chern numbers ±2 instead of the more common ±1. Similar topological phases could exist in dimer compounds such as Rb 2 Cu 3 SnF 12 (refs 46 , 47 ) with non-zero DM couplings, and possibly in ZnCu 3 (OH) 6 Cl 2 (Herbertsmithite) [48] . We predict a thermal Hall signature in SrCu 2 (BO 3 ) 2 that can be verified by transport measurements. We also suggest neutron scattering experiments to study the evolution of band structure in low-magnetic fields ( ≲ 2 T). Such measurements can see the spin-1 Dirac cone features at h z =0 and h z = h c . It may even be possible to directly probe the edge states using precise low-angle scattering measurements. How to cite this article : Romhányi, J. et al . Hall effect of triplons in a dimerized quantum magnet. Nat. Commun. 6:6805 doi: 10.1038/ncomms7805 (2015).